Single bunch X-ray pulses on demand from a multi-bunch synchrotron radiation source Synchrotron radiation facilities routinely operate in a multi-bunch regime, but applications relying on time-of-flight schemes require single bunch operation. Here we show that pulse picking by resonant excitation in a storage ring creates in addition to the multi-bunch operation a distinct and separable single bunch soft X-ray source. It has variable polarization, a photon flux of up to 10 7 –10 9 ph s −1 /0.1%BW at purity values of 10 4 –10 2 and a repetition rate of 1.25 MHz. The quasi-resonant excitation of incoherent betatron oscillations of electrons allows horizontal pulse separation at variable (also circular) polarization accessible for both, regular 30 ps pulses and ultrashort pulses of 2–3 ps duration. Combined with a new generation of angularly resolving electron spectrometers this creates unique opportunities for time-resolved photoemission studies as confirmed by time-of-flight spectra. Our pulse picking scheme is particularly suited for surface physics at diffraction-limited light sources promising ultimate spectral resolution. Synchrotron radiation (SR) research is driven by the rapid development of the source properties spectral brilliance, polarization and temporal definition in combination with X-ray’s unique capabilities to probe the atomic and electronic structure of matter in all aggregate states in an element-, chemical- and magnetic state selective manner. SR facilities worldwide are operated routinely at multi-bunch fill patterns for highest average brilliance since photon hungry experiments like X-ray diffraction, macromolecular crystallography, high resolution X-ray scattering and spectroscopy as well as X-ray microscopy benefit rather from maximum average brilliance of the source than it’s time structure. However, there is a highly innovative class of experiments that require kHz and few MHz pulsed SR for time-resolved or coincidence methods that enable conducting complete experiments in which all fragments of light-matter interaction are detected by time-of-flight (TOF) schemes. These requirements dictate to operate SR storage rings in dedicated single bunch mode shutting down effectively the majority of average brilliance experiments in multi-bunch operation. Hence, single bunch operation is provided by just a few facilities in the world and for very restricted times. A crucial objective is thus to operate SR storage rings and their beamlines in such a manner that each user may individually choose between single bunch and multi-bunch SR at each beamline and switch between these modes readily. Since the vertical emittance of SR storage rings is significantly smaller than the horizontal, the spectral monochromatization requires utilizing the vertical as the spectral dispersion plane. In consequence, the separation between multi- and single bunches should ideally utilize the orthogonal horizontal plane, although more challenging. In this work, we show how pulse picking by resonant excitation (PPRE) allows for separating photons from a single bunch horizontally, fully orthogonal to the dispersion planes, from the multi-bunch fill pattern. We verify the performance by TOF electron spectroscopy results. Before our work, vertical separation of single- and multibunch patterns has been shown at the advanced light source (ALS) [1] , [2] through a vertical kick-and-cancel scheme that generates a ‘pseudo-singlebunch’ at variable frequency by a vertical kicker in combination with a beamline that is capable of vertically separating photons emitted from a camshaft bunch that travels on a different closed orbit. The displacement varies from beamline to the next, depending on the location relative to the kicker that can operate from very low frequencies up to nearly the orbital revolution frequency [2] . Using the same method, first attempts at other facilities have been made [3] . A MHz pulse picking of a single bunch out of the multi-bunch fill pattern can be the pre-requisite to further downsample with kHz choppers [4] for ion spectroscopy and other slower applications. However, for realizing the dream of using separated photon pulses at the revolution frequency at any beamline of an existing light source on demand, we need to preserve, first of all, the vertical plane for spectral monochromatization. The larger angular/spatial horizontal separation then required is prohibitive to the existing kick-and-cancel scheme. We thus devised the PPRE scheme based on a combination of increased horizontal emittance of a single (camshaft or hybrid) bunch by a quasi-resonant incoherent excitation and a static local horizontal deflection of the electron beam that emits unwanted photons already upstream the beamline into a dump and only photons from the excited bunch into the beamline. The method involves static electron orbit manipulations in the range of fractions of mrad, while short- and long-term stability of the orbit is much lower and in the range of a few μrad. The stability of the quasi-resonant excitation of the incoherent betatron oscillation is also of the order of μrad t.e. some % of it's total amplitude. In addition, exactly the same blocking method has been successfully used over many years to horizontally separate X-rays from the time-sliced bunch at an elliptical insertion device at BESSY II [5] and at a planar undulator at the SLS [6] proving the stability of contemporary light sources sufficient for our purpose. Actually, the idea for the devised pulse picking scheme was initially based on these former experiences. PPRE provides an X-ray source ideally suited for high-resolution time-resolved photoelectron spectroscopy and we show the potential of this approach with angle-resolved time of flight (ARTOF) spectroscopy. Here, the Coulomb repulsion between all the emitted electrons on a sample’s surface sets a limit to the number of photons per X-ray pulse that can be used to reach a certain energy resolution [7] , [8] , [9] , and this number decreases with decreasing X-ray spot size and pulse duration. Peak brilliance is therefore not the main figure of merit for a high-resolution photoemission set-up. The performance is instead improved by increasing the repetition rate of the source and by optimizing the transmission of the spectrometer to accept a fraction of the emitted photoelectrons as large as possible. The angular-resolved TOF (ARTOF [10] , [11] ) provides this feature, combining outstanding transmission with high energy and angular resolution. The instrument also allows operation at a few MHz repetition rates, which is perfectly suited to the presented PPRE scheme. Here we show that the ARTOF instrument works very well with our new PPRE scheme, even when the storage ring is filled with ultrashort bunches at very low bunch currents. The ARTOF spectrometer and other time-resolved techniques have many attractive characteristics. All of these will benefit from the possibility to create single bunch radiation on demand at any undulator beamline during regular operation of the facility. Quasi-Resonant excitation of a single bunch The employed PPRE scheme is based on a quasi-resonant excitation of incoherent betatron oscillations of electrons in one particular bunch out of the entire temporal fill pattern. The light emitted from this bunch has a larger horizontal divergence than light emitted by bunches that are not excited. As illustrated in Fig. 1 , this particular beam property makes it possible to use a knife-edge aperture to pick only the X-ray pulses emitted by the excited bunch and block photons from the others. Note that the separation is achieved by moving the radiation of the unexcited beam horizontally away from the beam line’s axis with a closed orbit bump of the electron beam along the undulator. In this way, by using the on-axis radiation, we preserve the polarization properties of the picked photon beam pulse, even if emitted from an elliptical insertion device (like in the slicing case [4] ). If only one bunch, for example, a camshaft bunch in the clearing gap is selectively excited, the photon beam arriving at the experiment mimics a single electron bunch’s temporal emission pattern with 1.25 MHz repetition rate corresponding to the electron’s revolution time of 800 ns in the storage ring. The quasi-resonant excitation, however, has not to be done at 1.25 MHz but close to the horizontal betatron tune and corresponding sidebands of multiples of the revolution frequency. Therefore, and as explained below, a much lower frequency of ~190 kHz can be chosen, which leads to stationary but incoherent elongations of electrons at the revolution frequency of 1.25 MHz. 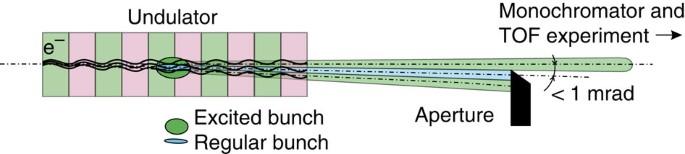Figure 1: Schematic illustration (view from above) of pulse picking by resonant excitation. Undulator light (blue) emitted from the regular electrons in other buckets (2 ns distance) is dumped into an aperture. In regular operation, the bump is turned off and the non-excited bunches (blue ellipse) emit undulator radiation on-axis. With the bump turned on, this radiation is emitted off-axis and hits the knife-edge being dumped there and only a part of the radiation from a resonantly excited (green) bunch can enter the beam line after travelling on-axis and thus, preserving the circular polarization degree (S3/S0)=0.7–0.9 as available from elliptical undulators. Figure 1: Schematic illustration (view from above) of pulse picking by resonant excitation. Undulator light (blue) emitted from the regular electrons in other buckets (2 ns distance) is dumped into an aperture. In regular operation, the bump is turned off and the non-excited bunches (blue ellipse) emit undulator radiation on-axis. With the bump turned on, this radiation is emitted off-axis and hits the knife-edge being dumped there and only a part of the radiation from a resonantly excited (green) bunch can enter the beam line after travelling on-axis and thus, preserving the circular polarization degree (S 3 /S 0 )=0.7–0.9 as available from elliptical undulators. Full size image The original pseudo-single bunch approach of the ALS [1] , [2] requires kicking the bunch on a turn-by-turn basis with always a similar angle, which is technically very challenging, especially in the horizontal plane. So far, only vertical kicks of <0.09 mrad with the necessary steep rise and fall times and the required repetition rate (~1 MHz) have been achieved. This approach provides single bunch capabilities at a few beamlines, which furthermore have to be individually adjusted to utilize the kicked beam at the experiment. The approach at BESSY is much different. In cases of many experiments (that is, TOF) where the full intensity of the bunch is not required, the following approach can be used: a typical bunch consists of a few times 10 10 electrons, which all perform transverse oscillations with frequencies spread around the so-called betatron tune. These oscillations are incoherent because the emission of SR by an electron is random and independent of the other electrons. The resulting excitation and damping process leads to a random distribution of phases and amplitudes of all individual oscillations and finally to a transverse Gaussian particle distribution. On the basis of our experience with emittance manipulation [12] , we use a quasi resonant excitation of the bunch to primarily blow up the beam horizontally. Only comparatively small kicks (<1 μrad) are required, and these small kicks add up more or less coherently and thus create a considerable increase in the horizontal beam size. Calculated photon flux curves are displayed in Fig. 2 as emitted by a 5 mA single bunch in an undulator at BESSY II for different electron beam emittances (see Supplementary Note 1 ). The vertical dashed line marks the position of a knife-edge aperture in the front end. With increased horizontal beam emittance, an increasing fraction of the light can pass through the aperture. A tenfold increase in the horizontal beam emittance (about a factor of 3 in divergence, see also Supplementary Note 2 and Supplementary Tables 1 and 2 ) is usually achieved with the excitation power levels used here. The undulator creates a light flash, albeit at lower intensity, every time the blown-up bunch passes by. As shown in Fig. 2 , it takes horizontal angles larger than 0.6 mrad to effectively separate the light produced by the excited single bunch from light emitted by the rest of the electrons. To preserve the polarization properties of the beam, the green part in Fig. 2 is horizontally kicked onto the beamline’s axis (0.0 mrad in Fig. 2 ) by a triangular local orbit manipulation described in Supplementary Fig. 1 and Supplementary Note 3 , which keeps the pulse-picked electrons on-axis along the undulator. Operating in the top-up-mode with such a blown-up bunch is possible if the excitation is turned off shortly before an injection takes place. Otherwise electrons of this bunch can get lost at the injection septum magnet. The blank-out pulse indicating an injection to the users ~20 ms in advance is used to suppress the excitation for 50 ms. This PPRE approach is fully compatible with user operation of BESSY II and already available on request. 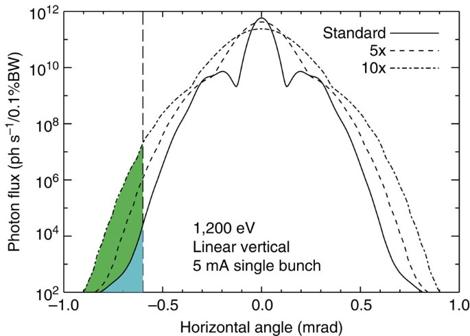Figure 2: Horizontal angular distribution of X-rays. Calculations of the horizontal flux distributions as emitted from a single bunch at 5 mA that passes the UE56 (Apple II) undulator at BESSY II. The solid line represents emission from standard operation. The dashed curves represent emission from resonantly excited bunches of fivefold and 10-fold increased effective emittance, respectively. It can be seen that accepting photons beyond a cut at about −0.6 mrad gives a high purity of up to 104for the PPRE radiation (green) that passes the aperture compared with the (blue) pedestal from the unexcited bunch. Figure 2: Horizontal angular distribution of X-rays. Calculations of the horizontal flux distributions as emitted from a single bunch at 5 mA that passes the UE56 (Apple II) undulator at BESSY II. The solid line represents emission from standard operation. The dashed curves represent emission from resonantly excited bunches of fivefold and 10-fold increased effective emittance, respectively. It can be seen that accepting photons beyond a cut at about −0.6 mrad gives a high purity of up to 10 4 for the PPRE radiation (green) that passes the aperture compared with the (blue) pedestal from the unexcited bunch. Full size image Regular user mode The PPRE method in the regular operation mode of the storage ring is demonstrated in Fig. 3 . Currently, the regular fill pattern of BESSY II contains four camshaft bunches in a 200 ns clearing gap as indicated by the fill pattern (blue) and signals from an Avalanche Photodiode (APD, negative record) behind the monochromator under the condition of the scheme drawn in Fig. 1 , but yet at rather weak excitation of the camshaft bunch that is in the centre of the clearing gap. Here, the aperture is set in a way to still detect some background signal ( Fig. 3a ) from the regular multi-bunch at an angular bump setting of −0.6 mrad. With PPRE switched on, under these conditions ( Fig. 3b ), the signal from the excited bunch considerably grows indicating that more photons pass the closed aperture. At another aperture setting (−0.65 mrad) and at three times higher amplitude of the quasi- resonant excitation, the core beam is completely suppressed ( Fig. 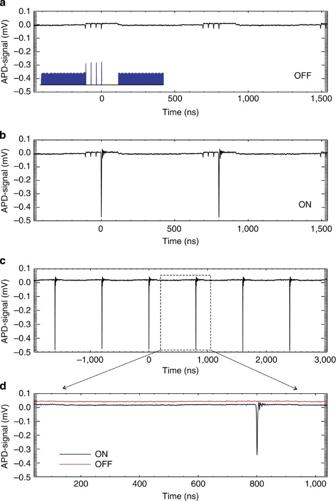Figure 3: X-ray signals at different excitation conditions. Signals as measured as avalanche photodiode (APD) signals (negative records) behind the exit slit of the UE56/1 beamline at a photon energy of 1,200 eV for different situations: (a) Normal hybrid mode with four camshaft bunches of mod (36 ns) distance in an ion clearing gap of 200 ns. The blue inset inashows the electron bunch structure (fill pattern). A weak resonant excitation of one camshaft bunch out of four inbleads already to one order of magnitude higher signal from that bunch. At even stronger excitation inc, a real stationary turn-by-turn repetition (shown by larger timescale) of the picked bunch at 800 ns (1.25 MHz) remains, even though the excitation is performed only at 190 kHz excitation frequency. A close-up of the single bunch signal inc, depicted indshows the result if the excitation is switched OFF and ON, respectively. The comparison between the black and the red curve (shifted for clarity) reveals that a signal contribution from multi-bunches is not detectable at all, even with a signal-to-noise limit >103. 3c ) and a single bunch X-ray signal of 10 7 –10 9 ph s −1 at 1.25 MHz (compare Supplementary Note 4 and Supplementary Table 3 ) at a purity of up to 10 2 –10 4 is detected that repeats stationary every 800 ns. The high purity is indicated by the complete disappearance of the signal if PPRE is switched off (red curve in Fig. 3d ). It should be mentioned here that a signal of >10 7 ph s −1 at 1.25 MHz is even approaching the maximum acceptable X-ray peak power level for very high-resolution PES on a micron-sized sample [7] . Figure 3: X-ray signals at different excitation conditions. Signals as measured as avalanche photodiode (APD) signals (negative records) behind the exit slit of the UE56/1 beamline at a photon energy of 1,200 eV for different situations: ( a ) Normal hybrid mode with four camshaft bunches of mod (36 ns) distance in an ion clearing gap of 200 ns. The blue inset in a shows the electron bunch structure (fill pattern). A weak resonant excitation of one camshaft bunch out of four in b leads already to one order of magnitude higher signal from that bunch. At even stronger excitation in c , a real stationary turn-by-turn repetition (shown by larger timescale) of the picked bunch at 800 ns (1.25 MHz) remains, even though the excitation is performed only at 190 kHz excitation frequency. A close-up of the single bunch signal in c , depicted in d shows the result if the excitation is switched OFF and ON, respectively. The comparison between the black and the red curve (shifted for clarity) reveals that a signal contribution from multi-bunches is not detectable at all, even with a signal-to-noise limit >10 3 . Full size image The PPRE method was also successfully tested with similar results at different undulators (UE52, UE56, U125) and at Spherical Grating (SGM) and Plane Grating (PGM)—monochromators [13] , respectively. Even at low photon energies down to 50 eV and up to 1,200 eV, a sufficiently clear separation of the single bunch pulses was always possible. Most promising was a first test there at the L -absorption edge of iron (~700 eV) in circular mode of the elliptical undulator indicating a feasibility of time-resolved magnetic experiments based on XMCD using photoelectron- or Auger electron detection. Low-α mode Bunch lengths of ~2–3 ps (r.m.s.) have been available for many years using BESSY II’s low-α mode [14] , [15] or even shorter bunches at lowest currents [16] . To test PPRE with ultra-short bunches, a special fill pattern with a bunch current of <100 μA of the camshaft bunch was created depicted by the blue curve in Fig. 4 . Albeit at somewhat less purity, the PPRE separation method applies here as well, as confirmed by the suppression of the multi-bunch APD-signal when blocking the regular beam more and more by the aperture ( Fig. 4a,b ). As it will become apparent below, this provides a roadmap for an excellent source of ps pulses at MHz repetition rates for ultrafast electron spectroscopy. 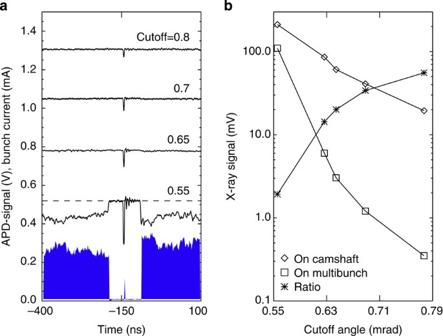Figure 4: X-ray signals in low-α mode under resonant excitation. X-ray signal as measured with an APD at the UE56/1 with PPRE for different cutoff angles. The envelope of the temporal current distribution in the storage ring as measured in the accelerator (blue curve ina) indicates the single bunch at <100 μA bunch current in the centre of a gap of 100 ns. The bunch is surrounded by a (non-uniform) pattern from the multi-bunch fill. The oscilloscope traces of the X-ray signal plotted in black inareflect different aperture settings (cutoff angles). The analysis of the measurements inbshows the peak signals for different aperture settings: squares—background signal from multi-bunch; diamonds—peak signal from the single bunch; black dots—purity (signal-over-background). Figure 4: X-ray signals in low-α mode under resonant excitation. X-ray signal as measured with an APD at the UE56/1 with PPRE for different cutoff angles. The envelope of the temporal current distribution in the storage ring as measured in the accelerator (blue curve in a ) indicates the single bunch at <100 μA bunch current in the centre of a gap of 100 ns. The bunch is surrounded by a (non-uniform) pattern from the multi-bunch fill. The oscilloscope traces of the X-ray signal plotted in black in a reflect different aperture settings (cutoff angles). The analysis of the measurements in b shows the peak signals for different aperture settings: squares—background signal from multi-bunch; diamonds—peak signal from the single bunch; black dots—purity (signal-over-background). Full size image Photoelectron spectroscopy We have successfully recorded photoelectron spectra employing the PPRE scheme using the newly developed ARTOF spectrometer. The ARTOF technique is based on the combination of an advanced electron lens with a two-dimensional time sensitive detector. The angular resolving mode of such a lens is based on the fact that the kinetic energy of the photoelectron and its take-off angles lead to a unique position at the focal plane at the end of the lens. However, the angular-resolved electrons are not projected on an entrance slit but hit the surface of a delay line detector. This detector measures the arrival time of the pulses and their x and y coordinates. Thus, we record in parallel the whole 2D angular pattern instead of only one angular coordinate. The kinetic energy of electrons can be recovered with a very high precision from the measured flight time in conjunction with the position on the detector [10] . A great advantage of the ARTOF type of electron analysers is the much higher acceptance, the resulting increased information rate in comparison with classical hemispherical analyzers and the much better resolution compared with classical TOF analysers [11] . The larger acceptance (about a factor of 10 3 ) compared to a hemispherical electron analyser more than compensates for the intensity loss due to our PPRE scheme. For the first proof of principle measurements with an ARTOF and our PPRE scheme in normal mode we used a Gold sample, the results are displayed in Fig. 5a,b . In the upper graph ( Fig. 5a ) one can clearly see mixed photoemission peaks exited by light from each of the four ‘camshaft’ bunches. However, as well known, the multi-bunch structure gives an additional high undesired background and mixed TOF traces from different bunches generally prohibit TOF experiments in multi-bunch operation of storage rings. When pulse picking is turned on as in Fig. 5b , a very clean TOF spectrum is seen proving that the picked pulse is clean enough to measure useful PES data. Another example experiment with PPRE switched ON and OFF is depicted in Fig. 5c,d , where the ring is operated in hybrid mode with only one camshaft pulse, but under low-α condition [15] . The clean spectrum in Fig. 5d reveals that, employing PPRE, one can get rid of the high background from the multibunch part as still seen in Fig. 5c . A useful electron kinetic energy spectrum like in Fig. 5d can be acquired in only a few minutes, even though the overall flux in the low-α mode is very small (see Supplementary Table 3 ) making it usually unfeasible to perform any kind of PES with hemispherical analysers. Pulse picking with our scheme reduces the flux compared with a dedicated single bunch mode, but due to the high angular acceptance of the ARTOF, it is no problem at all to acquire useful spectra even with weak ultrashort pulses. Here we work well below any space charge limits and time-resolved photoelectron spectroscopy experiments with picosecond time resolution at sub-meV energy resolution will soon come within reach. 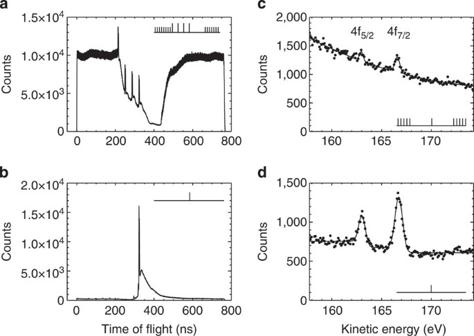Figure 5:Time-of-flight spectra from a Gold sample. Spectra as recorded with the ARTOF in regular user mode inaandband kinetic energy electron spectra taken in low—α mode from the same sample incanddunder different conditions. In the upper images (a) and (c) with PPRE OFF, spectra are contaminated by the multibunch part of the fill (see insets) showing that multibunch operation prohibits ARTOF experiments at all. On the contrary, clean spectra with PPRE ON can be measured inbanddif only light from the exited bunch arrives at the sample (see inset). Figure 5: Time-of-flight spectra from a Gold sample . Spectra as recorded with the ARTOF in regular user mode in a and b and kinetic energy electron spectra taken in low—α mode from the same sample in c and d under different conditions. In the upper images ( a ) and ( c ) with PPRE OFF, spectra are contaminated by the multibunch part of the fill (see insets) showing that multibunch operation prohibits ARTOF experiments at all. On the contrary, clean spectra with PPRE ON can be measured in b and d if only light from the exited bunch arrives at the sample (see inset). Full size image In summary, we have introduced a resonant pulse picking scheme, which allows us to separate X-ray pulses on demand from individual bunches in a storage ring filled with a multi-bunch fill pattern. The method is based on the quasi-resonant incoherent excitation of horizontal betatron oscillations of electrons in one particular bunch. The excitation leads to a selectively increased emittance of this particular bunch and causes a corresponding horizontal angular blurring of it’s undulator radiation cone. By deflecting the regular, very narrow unexcited part of the undulator radiation away from the beamline’s axis, only light from the excited bunch (at preserved polarization properties) can reach the experiment with a rate given by the revolution frequency (1.25 MHz). The set value of the local orbit bump ( Supplementary Fig. 1 ) together with slit positions in the beamline’s front end, that separate the useful photons, can be utilized to adapt different widths of the undulator radiation cone at different gap and shift settings [17] . Owing to this kind of separation, there is a loss of flux involved that, however, is acceptable and even mandatory for space charge limited photoemission experiments with modern highly transmitting end stations like the ARTOF. We have confirmed this by proof-of-principle experiments with an ARTOF instrument in different accelerator modes of BESSY II, at different undulators (UE56, UE52, U125) and at different beamlines: plane grating monochromators (PGM), zone plate monochromators (ZPM) and spherical grating monochromators (SGM). In case of elliptical insertion devices, the separation is possible even in the circular mode. Selecting light from ultrashort bunches and applications have also been performed in the so-called low-α mode of BESSY II with ultrashort pulses and at very low bunch currents of <100 μA. At last, and regardless of the operation mode, the user can select to use either the full static flux or alternatively to switch over within minutes to the ‘single bunch on demand’ situation without changing any other instrumental settings. Staying below space charge limits, the spectral resolution will be limited in future only by the vertical source size allowing for ultimate spectral resolution when combining diffraction limited (ultimate) storage rings, MHz pulse picking and TOF techniques. Electron bunch manipulation The electron bunch is kicked with the help of a stripline kicker. We use a dedicated kicker similar to the one of the transverse bunch-by-bunch feedback system. The kicker is powered by a 100 W-amplifier with a bandwidth ranging from 0.1 to 250 MHz. With the help of a ~5 ns long gate synchronized to the revolution frequency of 1.25 MHz, a signal is fed into the amplifier that thereby excites only the selected bunch in the ion-clearing gap. The frequency of the input signal is close to the lowest horizontal betatron resonance of 190 kHz and modulated in frequency over a few hundreds of Hz with a sweep frequency of 100 Hz. This together with the intrinsic tune spread among the electrons (created by wake fields and the energy and amplitude dependence of the tune) and the tune modulation of the resonance due to small mains ripples of the quadrupole gradients helps to excite the electrons as incoherently as possible. As a result, the centre of gravity oscillation of the bunch is much smaller than the blow-up of the beam size. The static horizontal orbit kick along the undulators to ensure on-axis light emission with preserved polarization from the pulse-picked electrons is described in Supplementary Fig. 1 and Supplementary Note 3 . Angle-resolved photoemission spectroscopy Angle-resolved photoelectron spectroscopy with pulse-picked X-rays was performed at BESSY II using the ARTOF instrument at the undulators UE56-1, UE52 and the U125. As monochromators, the plane grating monochromators (PGM) and spherical grating monochromators (SGM) were used at typical spectral resolution values of E/ΔE~5000. The Au 4 f spectra in Fig. 5 from the Gold sample at 160 meV analyser resolution were taken at a photon energy of 250 eV using the 1,200 l/mm grating and 100 μm slit at the UE56/1-PGM beam line. How to cite this article: Holldack, K. et al. Single bunch X-ray pulses on demand from a multi-bunch synchrotron radiation source. Nat. Commun. 5:4010 doi: 10.1038/ncomms5010 (2014).